TET2 repression by androgen hormone regulates global hydroxymethylation status and prostate cancer progression Modulation of epigenetic patterns has promising efficacy for treating cancer. 5-Hydroxymethylated cytosine (5-hmC) is an epigenetic mark potentially important in cancer. Here we report that 5-hmC is an epigenetic hallmark of prostate cancer (PCa) progression. A member of the ten–eleven translocation (TET) proteins, which catalyse the oxidation of methylated cytosine (5-mC) to 5-hmC, TET2, is repressed by androgens in PCa. Androgen receptor (AR)-mediated induction of the miR-29 family, which targets TET2, are markedly enhanced in hormone refractory PCa (HRPC) and its high expression predicts poor outcome of PCa patients. Furthermore, decreased expression of miR-29b results in reduced tumour growth and increased TET2 expression in an animal model of HRPC. Interestingly, global 5-hmC modification regulated by miR-29b represses FOXA1 activity. A reduction in 5-hmC activates PCa-related key pathways such as mTOR and AR . Thus, DNA modification directly links the TET2-dependent epigenetic pathway regulated by AR to 5-hmC-mediated tumour progression. Epigenetic processes regulate gene expression by altering the binding of transcription factors [1] . The DNA methylation pattern is an epigenetic code that defines the global gene regulatory state [2] . The resultant regulation of gene expression is thought to govern various biological phenomena, including cancer progression. 5-Hydroxymethylation of cytosine bases (5-hmC) is a newly identified epigenetic marker; this nontraditional DNA modification involves methylation of cytosine bases (5-mC) in CpG dinucleotide sequences [2] , [3] and their oxidation by the ten–eleven translocation (TET) family of proteins. While 5-hmC is a potentially useful indicator of disease states such as cancer [4] , [5] , [6] , [7] , [8] , the mechanisms controlling its abundance in tumours and its impact on gene expression and cancer cell fate are unclear. Androgen receptor (AR) signalling is crucial for prostate tumour growth [9] , [10] , [11] , [12] , [13] . When bound to androgens, ARs translocate to the nucleus and transactivate target genes by interacting with other transcription factors such as forkhead-box A1 (FOXA1) [10] . Although the molecular mechanisms underlying prostate cancer progression to lethal hormone refractory prostate cancer (HRPC) [9] , [10] , [11] , [12] , [13] are incompletely understood, activation of downstream signals by hypersensitive or overexpressed ARs is considered to be important. The epigenetic status of prostate cancer cells is modulated by AR binding and the subsequent recruitment of co-activators or co-repressors [14] , [15] , [16] , [17] , [18] . Acetylation, methylation, phosphorylation, ubiquitylation and ADP ribosylation of histones critically affect transcriptional regulation by ARs [19] , [20] , [21] . The main epigenetic mechanism that controls AR binding to DNA in prostate cancer is histone modification by histone acetyltransferases, histone methyltransferases and protein kinases at AR-binding sites (ARBSs) [20] , [21] . Specific epigenetic codes modulate opening of chromatin to induce or repress the expression of protein-encoding genes and non-coding RNAs [11] . The relationship between AR activity and DNA modifications, particularly 5-mC hydroxylation, has not been described previously, and the role of androgen-targeted non-coding RNAs such as micro RNAs (miRNAs) in global epigenetic control is largely unknown. Here we report that 5-hmC is an epigenetic hallmark of prostate cancer inversely associated with disease progression. We show that AR-induced miRNA represses the expression of a member of the TET family, TET2, and that low expression levels of TET2 are correlated with low 5-hmC levels in advanced clinical tumours. Global mapping indicated that hydroxylation of 5-mC suppressed FOXA1 enhancer activity and impacted on prostate cancer-related pathways such as the AR pathway. Our findings suggest that AR-modulated TET2 pathways form the basis of a new treatment strategy for advanced, HRPCs. TET2 is repressed by androgens in prostate cancer cells We established bicalutamide (AR antagonist)-resistant prostate cancer (BicR) cells derived from an AR-positive, bicalutamide-sensitive LNCaP prostate cancer cell line ( Supplementary Fig. 1a ). We first examined the androgen-regulated signals in both BicR and LNCaP cells, and the differences between them using AR chromatin immunoprecipitatio sequence (ChIP-seq) and cap analysis of gene expression (CAGE) [22] , [23] , a powerful tool for analysing global transcriptome. Interestingly, ARBSs obtained by bicalutamide treatment in BicR cells overlap with those by AR agonist, dihydrotestosterone (DHT), treatment, suggesting that bicalutamide mediates AR recruitment to the genomic regions ( Supplementary Fig. 1b ). 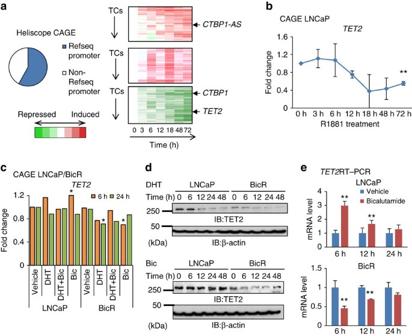Figure 1: TET2 is differentially regulated by androgen in hormone-dependent and hormone refractory prostate cancer. (a) To analyse the androgen-regulated transcriptional program, we prepared total RNA extracted from LNCaP cell lines treated with 10 nM R1881 at seven time points in each biological duplicate.CTBP1andCTBP1-ASare positive control androgen-regulated genes49. (b)TET2is repressed by R1881 10-nM treatment in LNCaP cells. Time course of CAGE data (fold induction); duplicate biological samples were evaluated at each time point. Values represent the mean±s.d. **P<0.01 (two-sided Student’st-test). (c) Regulation ofTET2, as determined by CAGE, in LNCaP and BicR cells treated with vehicle, 10 nM DHT, 10 nM DHT+1 μM bicalutamide or 1 μM bicalutamide for 6 or 24 h.Pvalue is determined by Fisher’s exact test. (d) Immunoblots (IBs) of extracts from LNCaP and BicR cells treated with 10 nM DHT or 1 μM bicalutamide for the indicated time. (e) Regulation ofTET2mRNA expression by bicalutamide in LNCaP and BicR cells. Both cell lines were treated with vehicle or bicalutamide for 6, 12 or 24 h.TET2mRNA induction was measured by qRT–PCR (n=3). Values represent the mean±s.d. *P<0.05, **P<0.01 (two-sided Student’st-test). In addition, we also explored androgen-induced miRNAs by sequence analysis of comprehensive short RNA profiles ( Supplementary Table 1 ; Supplementary Fig. 2a ) to analyse the role of miRNA in prostate cancer progression. In LNCaP cells, a total of 44 miRNAs were significantly induced by DHT (>1.2-fold), including representative AR-regulated miRNAs such as miR-125b [24] , miR-21 (ref. 25 ) and miR-148a [26] , while 30 miRNAs were induced by DHT (>1.2-fold) in BicR cells. The members of the miR-29 family and miR-22 were the most responsive to androgen treatment in BicR cells compared with parental LNCaP cells. Our in silico analysis of their direct target raised the possibility that both miRNAs target TET2 , one of the key epigenetic regulatory factors ( Supplementary Fig. 2b ). Next, our investigation of R1881 (AR agonist)-regulated genes in LNCaP cells ( Fig. 1a ) using CAGE showed that TET2 was repressed by androgen treatment ( Fig. 1b ). To further investigate the androgen signalling during prostate cancer progression, we also performed CAGE in both LNCaP and BicR cells treated with vehicle, DHT or bicalutamide. We identified 243 and 256 promoters that were upregulated by more than twofold by DHT in LNCaP and BicR cells, respectively. Among these promoters, 66 were commonly regulated in both cell lines, while the others were cell-type specific ( Supplementary Fig. 1c ). LNCaP-specific promoters were upregulated without DHT treatment in BicR cells, indicating androgen hypersensitivity in these cells ( Supplementary Fig. 1d ). In BicR-specific promoters, androgen-dependent activation is more evident in BicR cells than in LNCaP cells ( Supplementary Fig. 1e ). We then found that negative regulation of TET2 by DHT and bicalutamide was more evident in BicR cells than in LNCaP cells ( Fig. 1c ). TET2 was upregulated by bicalutamide treatment and downregulated by DHT treatment in LNCaP cells, while it was downregulated by both DHT and bicalutamide in BicR cells ( Fig. 1d,e ; Supplementary Fig. 3a ). Figure 1: TET2 is differentially regulated by androgen in hormone-dependent and hormone refractory prostate cancer. ( a ) To analyse the androgen-regulated transcriptional program, we prepared total RNA extracted from LNCaP cell lines treated with 10 nM R1881 at seven time points in each biological duplicate. CTBP1 and CTBP1-AS are positive control androgen-regulated genes [49] . ( b ) TET2 is repressed by R1881 10-nM treatment in LNCaP cells. Time course of CAGE data (fold induction); duplicate biological samples were evaluated at each time point. Values represent the mean±s.d. ** P <0.01 (two-sided Student’s t -test). ( c ) Regulation of TET2 , as determined by CAGE, in LNCaP and BicR cells treated with vehicle, 10 nM DHT, 10 nM DHT+1 μM bicalutamide or 1 μM bicalutamide for 6 or 24 h. P value is determined by Fisher’s exact test. ( d ) Immunoblots (IBs) of extracts from LNCaP and BicR cells treated with 10 nM DHT or 1 μM bicalutamide for the indicated time. ( e ) Regulation of TET2 mRNA expression by bicalutamide in LNCaP and BicR cells. Both cell lines were treated with vehicle or bicalutamide for 6, 12 or 24 h. TET2 mRNA induction was measured by qRT–PCR ( n =3). Values represent the mean±s.d. * P <0.05, ** P <0.01 (two-sided Student’s t -test). Full size image TET2 is a key target gene of androgen-regulated miRNAs To examine the roles of the androgen-regulated miRNAs in TET2 regulation, we transfected the cells with miRNA mimics and a luciferase vector containing the 3′ untranslated region (UTR) sequence of TET2. Consequently, miR-125b, miR-22, miR-30a, miR-200a and miR-29a/b were found to repress the luciferase activity, suggesting the possibility of TET2 repression by androgen-regulated miRNAs ( Fig. 2a ). Notably, among all androgen-regulated miRNAs tested, miR-29a/b repressed the luciferase activity most strikingly. As suggested by the sequence analysis, miR-29a/b was markedly overexpressed and highly responsive to androgen in BicR cells compared with LNCaP cells ( Fig. 2b ). We observed that primary miR-29a/b1 transcript was induced by DHT, although pri-miR-29b2 was not ( Supplementary Fig. 3b ). Then, ARBSs were found around the miR-29a/b1 locus by AR ChIP-seq analysis in LNCaP and BicR cells ( Fig. 2c ; Supplementary Fig. 3c ). Using bioinformatics, we identified the enrichment of four potential miR-29-family-binding sites in the 3′UTR sequence of TET2 ( Fig. 2a ). We also demonstrated that the repression of TET2 by miR-29a/b is dependent on these sites ( Fig. 2d ; Supplementary Fig. 3d ), while the downregulation of miR-29a/b enhances the expression level of the TET2 protein ( Fig. 2e ; Supplementary Fig. 3e,f ). Conversely, the overexpression of miR-29a/b was found to repress TET2 expression ( Fig. 2f ). In addition, the gain and loss of miR-29a/b expression are associated with the level of 5-hmC, but not 5-mC, in prostate cancer cells ( Supplementary Figs 3g and 4a ). Although most AR-positive castration-resistant prostate cancer (CRPC) cell lines such as long-term androgen deprivation (LTAD) cells exhibit low levels of TET2 expression, the inhibition of miR-29a/b by anti-miR-29a/b transfection increased the TET2 expression and reversed DHT-mediated TET2 repression ( Supplementary Fig. 4b–d ). 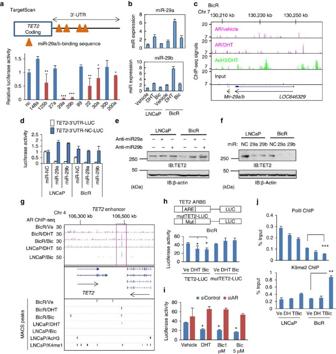Figure 2: Mechanism of TET2 repression by androgen-regulated miRNAs and AR in HRPC. (a) Upper:TET23EUTR including miR-29-binding sequences. Lower: a luciferase vector including theTET23EUTR and several mimics of androgen-regulated miRNAs were transfected into LNCaP cells; 48 h after transfection, cells were lysed and a luciferase assay was performed (n=3). Values represent the mean±s.d. *P<0.05, **P<0.01, ***P<0.001 (two-sided Student’st-test). (b) qRT–PCR of miR-29a/b in LNCaP and BicR cells was performed. Cells were treated with vehicle, 10 nM DHT and 1 μM bicalutamide for 24 h. (n=3). Values represent the mean±s.d. (c) Mapping of AR-binding sites in the vicinity of themiR-29a/b1locus. The black arrow shows the direction of miRNAs. (d) LNCap and BicR cells were transfected with luciferase vectors TET2-3′UTR and TET2-3′UTR-NC, with control miR (NC) or miR-29a/b. (n=3). Values represent the mean±s.d. (e) Immunoblot (IB) of cell lysates from LNCaP and BicR cells transfected with anti-miRNA-29a/b to detect TET2 protein levels. (f) Immunoblots of cell lysates of LNCaP and BicR cells transfected with miRNA-29a/b to detect TET2 protein levels. (g) Mapping of AR-binding sites in the vicinity of theTET2locus. The black arrow shows the direction of genes. The red box indicates the TET2-enhancer region. (h) A luciferase vector including theTET2enhancer region with or without mutated androgen response elements was transfected into BicR cells. Cells were treated with vehicle, 10 nM DHT or 1 μM bicalutamide for 24 h, and then a luciferase assay was performed (n=3). Values represent the mean±s.d. *P<0.05 (two-sided Student’st-test). (i) A luciferase vector including TET2-enhancer region was transfected into BicR cells, which were treated with siControl or siAR (10 nM) for 48 h. Cells were treated with vehicle, 10 nM DHT or bicalutamide (1 or 5 μM) for 24 h and then luciferase activity was measured (n=3). Values represent the mean±s.d. ***P<0.001 (two-sided Student’st-test). (j) ChIP analysis of K9me2 and Pol II in theTET2-enhancer region in LNCaP and BicR cells were treated with vehicle, 10 nM DHT or 1 μM bicalutamide for 24 h. Enrichment over input (% input) was measured by qPCR (n=3). Values represent the mean±s.d. **P<0.01 (two-sided Student’st-test). Figure 2: Mechanism of TET2 repression by androgen-regulated miRNAs and AR in HRPC. ( a ) Upper: TET2 3EUTR including miR-29-binding sequences. Lower: a luciferase vector including the TET2 3EUTR and several mimics of androgen-regulated miRNAs were transfected into LNCaP cells; 48 h after transfection, cells were lysed and a luciferase assay was performed ( n =3). Values represent the mean±s.d. * P <0.05, ** P <0.01, *** P <0.001 (two-sided Student’s t -test). ( b ) qRT–PCR of miR-29a/b in LNCaP and BicR cells was performed. Cells were treated with vehicle, 10 nM DHT and 1 μM bicalutamide for 24 h. ( n =3). Values represent the mean±s.d. ( c ) Mapping of AR-binding sites in the vicinity of the miR-29a/b1 locus. The black arrow shows the direction of miRNAs. ( d ) LNCap and BicR cells were transfected with luciferase vectors TET2-3′UTR and TET2-3′UTR-NC, with control miR (NC) or miR-29a/b. ( n =3). Values represent the mean±s.d. ( e ) Immunoblot (IB) of cell lysates from LNCaP and BicR cells transfected with anti-miRNA-29a/b to detect TET2 protein levels. ( f ) Immunoblots of cell lysates of LNCaP and BicR cells transfected with miRNA-29a/b to detect TET2 protein levels. ( g ) Mapping of AR-binding sites in the vicinity of the TET2 locus. The black arrow shows the direction of genes. The red box indicates the TET2-enhancer region. ( h ) A luciferase vector including the TET2 enhancer region with or without mutated androgen response elements was transfected into BicR cells. Cells were treated with vehicle, 10 nM DHT or 1 μM bicalutamide for 24 h, and then a luciferase assay was performed ( n =3). Values represent the mean±s.d. * P <0.05 (two-sided Student’s t -test). ( i ) A luciferase vector including TET2-enhancer region was transfected into BicR cells, which were treated with siControl or siAR (10 nM) for 48 h. Cells were treated with vehicle, 10 nM DHT or bicalutamide (1 or 5 μM) for 24 h and then luciferase activity was measured ( n =3). Values represent the mean±s.d. *** P <0.001 (two-sided Student’s t -test). ( j ) ChIP analysis of K9me2 and Pol II in the TET2 -enhancer region in LNCaP and BicR cells were treated with vehicle, 10 nM DHT or 1 μM bicalutamide for 24 h. Enrichment over input (% input) was measured by qPCR ( n =3). Values represent the mean±s.d. ** P <0.01 (two-sided Student’s t -test). Full size image AR directly represses TET2-enhancer activity in HRPC To elucidate the mechanism of TET2 repression by bicalutamide in BicR cells, we examined the possibility that TET2 is directly regulated by AR. Using ChIP-seq analysis, we found that AR was recruited to the distal enhancer region of TET2 by DHT treatment in both cell lines. Interestingly, after bicalutamide treatment, AR binding could be detected in the enhancer region only in BicR cells ( Fig. 2g ; Supplementary Fig. 4e ). Unlike typical ARBSs, this locus does not mediate positive transcriptional activity in response to DHT treatment. Moreover, the bicalutamide-mediated repression of the enhancer activity in BicR cells is dependent on androgen response elements in the middle of the ARBS ( Fig. 2h,i ). ChIP analysis indicated that this enhancer is directly repressed by repressive histone modification (increased levels of histone H3K9 methylation) in the antagonist-bound condition ( Fig. 2j ; Supplementary Fig. 4f ). In addition, chromatin conformational capture (3C) assay was performed to show the physical interaction of promoter/enhancer in the TET2 locus ( Supplementary Fig. 5 ). We found that the long-range interaction was significantly enhanced in BicR cells compared with LNCaP cells. In addition, 3C–ChIP products were immunoprecipitated by AR antibody, showing that the chromatin conformation at the TET2 locus was changed by the complex, including AR. This result is compatible with our other analyses suggesting the direct regulation of TET2 by AR in BicR. Thus, in bicalutamide-treated HRPC cells, both indirect miR-dependent regulation and direct AR-mediated repression are important in TET2 repression. Clinical significance of TET2 repression in prostate cancer To investigate the role of TET2 and its associated epigenetic marker, 5-hmC, in prostate cancer progression, we evaluated the levels of TET2 and 5-hmC in clinical tumour samples by immunohistochemistry ( Fig. 3a ). Strong nuclear 5-hmC staining was observed in benign prostate tissues surrounding the tumours, whereas partial or complete reduction of 5-hmC staining was observed in a subset of tumour samples. Interestingly, decreased expression of TET2 and 5-hmC could be a prognostic factor predicting the survival of patients after surgery ( Fig. 3b,c ). Low expression level of TET2 is not associated with Gleason scores, but with metastasis or advanced stages of cancer ( Supplementary Table 2 ). 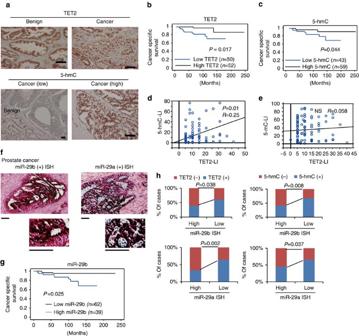Figure 3: Clinical significance of miR-29 family and TET2 protein expression in prostate cancer. (a) TET2 and 5-hmC are downregulated in a subset of prostate cancer samples. Immunohistochemistry of 5-hmC and TET2 in prostate cancer and benign prostate tissues (n=102) was performed. Scal, bar, 100 μm. (b,c) Downregulation of TET2 (b) and 5-hmC (c) is a prognostic factor for prostate cancer. Kaplan–Meier analysis using the log-rank test was performed. (d) Positive correlation of TET2 expression with 5-hmC levels. (e) No significant correlation between 5-mC and TET2 expression levels. Regression analysis was performed to analyse the correlation. NS, not significant. (f) miR-29 expression levels were analysed byin situhybridization (ISH) in prostate cancer samples (n=101). Scale bar, 100 μm. (g) High miR-29b expression is a prognostic factor for prostate cancer patients. Kaplan–Meier analysis using the log-rank test was performed. (h) The association of miR-29 a/b with 5-hmC level and TET2 protein level was analysed by theχ2-test. Importantly, we found that TET2 repression is an independent prognostic factor by multivariate analysis ( Supplementary Table 3 ). Using publicly available microarray data sets (GSE3325, GSE6919 and GSE35988) of prostate cancer clinical samples, we confirmed that TET2 expression is significantly repressed in metastatic prostate cancer compared with localized tumours ( Supplementary Fig. 7a ). Thus, these results indicate that TET2 repression is associated with disease progression, in particular, metastasis. In contrast, strong 5-mC staining is present in both the cancerous and normal prostate tissues ( Supplementary Fig. 6a ). We also confirmed the positive correlation of TET2 expression with 5-hmC but not 5-mC ( Fig. 3d,e ). These findings suggest that deceased expression of both 5-hmC and TET2 represent a new epigenetic marker associated with survival rate and tumour progression of prostate cancer patients. Figure 3: Clinical significance of miR-29 family and TET2 protein expression in prostate cancer. ( a ) TET2 and 5-hmC are downregulated in a subset of prostate cancer samples. Immunohistochemistry of 5-hmC and TET2 in prostate cancer and benign prostate tissues ( n =102) was performed. Scal, bar, 100 μm. ( b , c ) Downregulation of TET2 ( b ) and 5-hmC ( c ) is a prognostic factor for prostate cancer. Kaplan–Meier analysis using the log-rank test was performed. ( d ) Positive correlation of TET2 expression with 5-hmC levels. ( e ) No significant correlation between 5-mC and TET2 expression levels. Regression analysis was performed to analyse the correlation. NS, not significant. ( f ) miR-29 expression levels were analysed by in situ hybridization (ISH) in prostate cancer samples ( n =101). Scale bar, 100 μm. ( g ) High miR-29b expression is a prognostic factor for prostate cancer patients. Kaplan–Meier analysis using the log-rank test was performed. ( h ) The association of miR-29 a/b with 5-hmC level and TET2 protein level was analysed by the χ 2 -test. Full size image Using in situ hybridization (ISH), we demonstrated that miR-29a/b expression in clinical prostate cancer tissues ( Fig. 3f ; Supplementary Fig. 6b ) is associated with poor prognosis ( Fig. 3g ; Supplementary Fig. 6c ). We also observed that the expression of the miR-29 family is negatively correlated with that of TET2 and 5-hmC ( Fig. 3h ). Furthermore, quantitative PCR with reverse transcription (qRT–PCR) analysis of miR-29b and TET2 expression in clinical samples of prostate cancer obtained by laser capture microdisection is in line with ISH results ( Supplementary Fig. 6d,e ). Furthermore, in a public microarray data set (GSE21036 and GSE21034), we found that upregulation of miR-29a/b and repression of TET2 in advanced prostate cancer samples ( Supplementary Fig. 7b–d ). In other cohorts (GSE45604, GSE23022 and GSE46738), we also observed that high miR-29a/b expressions are associated with high Gleason scores, as observed in our ISH study ( Supplementary Fig. 7e,f ; Supplementary Tables 4 and 5 ). Taken together, our results suggest that miR-29-mediated TET2 repression for 5-hmC inhibition is a mechanism involved in prostate cancer progression. TET2-related pathway is responsible for tumour growth We next determined whether TET2 repression is associated with tumour growth. We first performed proliferation assays in LNCaP and BicR cells and demonstrated that the overexpression and knockdown of miR-29a/b increased and decreased the proliferation of LNCaP cells, respectively ( Supplementary Fig. 8a–c ). Importantly, inhibition of cell growth by anti-miR-29a/b was significant in antagonist-treated BicR cells ( Fig. 4a ). To investigate whether this effect of miRNA is mediated by TET2 repression, we overexpressed TET2 in VCaP cells and knocked down TET2 expression in LNCaP cells by transfections with a TET expression vector or short interfering RNA (siRNA) targeting TET2 , respectively ( Fig. 4b ). The gain or loss of TET2 expression had a significant effect on cell proliferation ( Fig. 4c,d ), demonstrating the growth inhibitory effect of TET2 in prostate cancer. We also demonstrated that TET2 growth inhibitory ability was associated with the C-terminal domain important for its enzymatic activity [27] ( Supplementary Fig. 9 ). In addition, miR-29b-mediated induction of cell proliferation was abrogated by the rescue of TET2 expression ( Fig. 4e ), while anti-miR-29b-mediated inhibition of cell growth was relieved by TET2 knockdown ( Fig. 4f ). Moreover, miR-29a/b was positively regulated by AR and promoted cell growth in other prostate cancer cells (DU145 and VCaP cells; Supplementary Fig. 8d–i ). To examine the role of miR-29a/b and TET2 in castration resistance, we also transfected CRPC cell lines with anti-miR-29a/b and observed a repression of castration-resistant cell growth ( Supplementary Fig. 10 ). Notably, cell migration was markedly enhanced in BicR cells compared with parental LNCaP cells ( Supplementary Fig. 11a ). Transfection of the BicR cells with anti-miR-29b reduced cell migration, suggesting that miR-29b induction promotes BicR cell migration by repressing TET2 ( Fig. 4g ). Taken together, these results indicate that the miR-29 family has a tumour-promoting effect in prostate cancer. 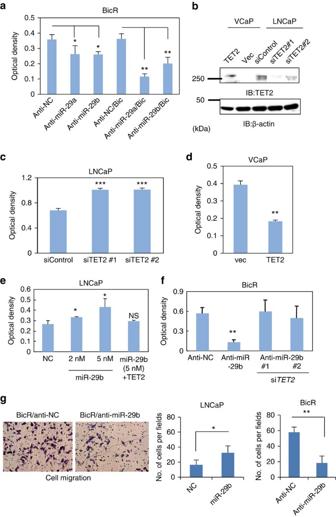Figure 4: Critical role of miR-29a/b and TET2 repression for hormone refractory prostate cancer cell growth and migration. (a) Growth of BicR cells in medium with or without 10 μM bicalutamide after transfection of anti-negative control (anti-NC) or anti-miR-29a/b (n=4). Values represent the mean±s.d. *P<0.05, **P<0.01 (two-sided Student’st-test). (b) Expression levels of TET2 protein level by western blot analysis. VCaP cells were transfected with an empty vector or TET2 expression vector. LNCaP cells were transfected with siControl, siTET2#1 or siTET2#2 (1 nM). (c) Growth of LNCaP cells transfected with siControl, siTET2#1 or siTET2#2 (1 nM;n=4). Values represent the mean±s.d. ***P<0.001 (two-sided Student’st-test). (d) Growth of VCaP cells transfected with TET2 expression vector or control vector (n=4). Values represent the mean±s.d. **P<0.01 (two-sided Student’st-test). (e) Growth of LNCaP cells transfected with miR-29b with or without rescue of TET2 (n=4). Values represent the mean±s.d. *P<0.05 (two-sided Student’st-test). (f) Growth of BicR cells transfected with anti-miR-29b with or without knockdown of TET2 (n=4). Values represent the mean±s.d. **P<0.01 (two-sided Student’st-test). (g) LNCaP and BicR cells were seeded onto filters with an 8 μm pore size in a matrigel-coated upper chamber. The average numbers of invading cells per field are shown (n=5). Cells were treated with miR-29b or anti-miR-29b. Values represent the mean±s.d. *P<0.05, **P<0.01 (two-sided Student’st-test). IB, immunoblot. Figure 4: Critical role of miR-29a/b and TET2 repression for hormone refractory prostate cancer cell growth and migration. ( a ) Growth of BicR cells in medium with or without 10 μM bicalutamide after transfection of anti-negative control (anti-NC) or anti-miR-29a/b ( n =4). Values represent the mean±s.d. * P <0.05, ** P <0.01 (two-sided Student’s t -test). ( b ) Expression levels of TET2 protein level by western blot analysis. VCaP cells were transfected with an empty vector or TET2 expression vector. LNCaP cells were transfected with siControl, si TET2 #1 or si TET2 #2 (1 nM). ( c ) Growth of LNCaP cells transfected with siControl, si TET2 #1 or si TET2 #2 (1 nM; n =4). Values represent the mean±s.d. *** P <0.001 (two-sided Student’s t -test). ( d ) Growth of VCaP cells transfected with TET2 expression vector or control vector ( n =4). Values represent the mean±s.d. ** P <0.01 (two-sided Student’s t -test). ( e ) Growth of LNCaP cells transfected with miR-29b with or without rescue of TET2 ( n =4). Values represent the mean±s.d. * P <0.05 (two-sided Student’s t -test). ( f ) Growth of BicR cells transfected with anti-miR-29b with or without knockdown of TET2 ( n =4). Values represent the mean±s.d. ** P <0.01 (two-sided Student’s t -test). ( g ) LNCaP and BicR cells were seeded onto filters with an 8 μm pore size in a matrigel-coated upper chamber. The average numbers of invading cells per field are shown ( n =5). Cells were treated with miR-29b or anti-miR-29b. Values represent the mean±s.d. * P <0.05, ** P <0.01 (two-sided Student’s t -test). IB, immunoblot. Full size image We further analysed the downstream signals of miR-29b and TET2 in LNCaP cells. The overexpression of miR-29b and knockdown of TET2 induced the expression of 495 genes, suggesting that these genes are putative targets of TET2 ( Supplementary Fig. 12a ). Gene ontology (GO) term analysis for these genes showed that they are significantly involved in cell migration ( Supplementary Fig. 12b ). In addition to the TET2 downstream signalling, microarray and GO term analysis suggested that miR-29b significantly induces cell cycle-related pathway such as Aurora kinase A ( AURKA ), which is involved in the miR-29a/b-mediated growth promotion ( Supplementary Figs 12c and 13a,b,d–g ). Furthermore, although our comprehensive analysis of miR-29a/b targets revealed that TET2 is the primary target of miR-29a/b in prostate cancer cells ( Supplementary Fig. 12d,e ), HMG-box transcription factor 1 ( HBP1 ), a tumour suppressor gene [28] , was identified as another miR-29b direct target in LNCaP cells for cell proliferation ( Supplementary Fig. 13c,h,i ). Thus, although TET2 is the major determinant of miR-29 downstream signalling, cooperative functions of these activated pathways or target genes would be associated with miR-29b-mediated growth promotion. Next, we examined the roles of miR-29b and TET2 in tumour progression using in vivo xenograft assays. Nude mice were injected with LNCaP or BicR cells and monitored for tumour growth. Oral bicalutamide treatment inhibited LNCaP tumour growth ( Supplementary Fig. 11b ), but not BicR tumour growth. However, anti-miR-29b injections (three times a week) into the BicR tumours significantly inhibited the tumour growth ( Fig. 5a,b ). Importantly, TET2 expression was higher in the tumours treated with anti-miR-29b than in the control BicR tumours, even in the presence of bicalutamide ( Fig. 5c,d ). Furthermore, we also demonstrated that repression of miR-29a/b inhibited castration-resistant tumour growth in xenografts of CRPC cell lines (22Rv1 and LTAD cells; Supplementary Fig. 14 ). Taken together, these data highlight a potential role of increased miR-29-family-mediated TET2 repression in the progression of prostate cancer to HRPC. 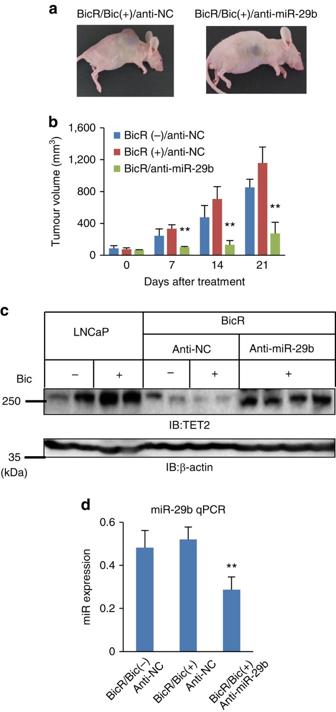Figure 5: Hormone refractory tumour growth is inhibited by modulating miR-29 and TET2 pathway. (a) Nude mice were inoculated with BicR cells; tumour growth (b) of xenografted BicR cells in nude mice treated with anti-NC or anti-miR-29b are shown (n=7). Values represent the mean±s.d. **P<0.01 (two-sided Student’st-test). Vehicle or bicalutamide was administered orally each day. Representative views of tumours in nude mice are shown. (c) Western blot analysis was performed to evaluate TET2 expression levels in tumours (n=2). (d) Downregulation of miR-29b in tumour cells injected with anti-miR-29b (n=4). qRT–PCR was performed to measure the miRNA expression level in those tumours. Values represent the mean±s.d. **P<0.01 (two-sided Student’st-test). IB, immunoblot. Figure 5: Hormone refractory tumour growth is inhibited by modulating miR-29 and TET2 pathway. ( a ) Nude mice were inoculated with BicR cells; tumour growth ( b ) of xenografted BicR cells in nude mice treated with anti-NC or anti-miR-29b are shown ( n =7). Values represent the mean±s.d. ** P <0.01 (two-sided Student’s t -test). Vehicle or bicalutamide was administered orally each day. Representative views of tumours in nude mice are shown. ( c ) Western blot analysis was performed to evaluate TET2 expression levels in tumours ( n =2). ( d ) Downregulation of miR-29b in tumour cells injected with anti-miR-29b ( n =4). qRT–PCR was performed to measure the miRNA expression level in those tumours. Values represent the mean±s.d. ** P <0.01 (two-sided Student’s t -test). IB, immunoblot. Full size image 5-hmC plays a critical role in FOXA1 enhancer activity We next explored whether loss of 5-hmC in prostate cancer is genome wide or locus specific using chemical labelling (biotinylation) of 5-hmC and subsequent immunoprecipitation with streptavidin beads (5-hmC collector) [29] . We coupled this approach with deep sequencing using a ChIP-seq protocol. This assay permits quantitative comparisons of genome-wide changes in 5-hmC levels between cell lines. Using model-based analysis of ChIP-seq (MACS) [30] , we determined global 5-hmC regions ( P value<10 −5 , Poisson distribution, false discovery rate (FDR)<0.01; Fig. 6a ) in prostate cancer cells. Interestingly, although the number of 5-hmC sites was reduced in BicR cells compared with LNCaP cells, as expected from the decrease of TET2 expression, the inhibition of miR-29b markedly increased the number of 5-hmC sites ( Fig. 6a , top panel). We also performed another assay, hMedIP, and confirmed that 5-hmC levels were repressed in BicR cells compared with LNCaP cells ( Fig. 6b ). Moreover, the 5-hmC regions appeared to overlap with the 5-mC regions, due to the generation of 5-hmC by the oxidation of 5-mC ( Fig. 6c ). 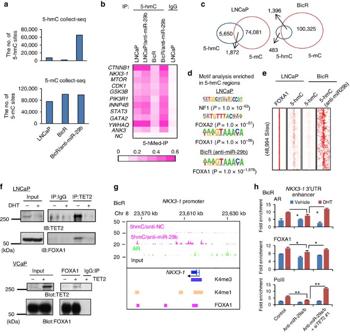Figure 6: Global analysis of 5-hmC-regulated pathways in prostate cancer progression. (a) Global mapping of genomic regions modified with 5-hmC (upper) and 5-mC (lower) in prostate cancer cells. Genomic DNA was extracted from LNCaP cells and from BicR cells treated with anti-NC or anti-miR-29b. Binding regions were determined by MACS. (b) Validation of 5-hmC levels in LNCaP and BicR cells by hMeDIP. Cells were transfected with anti-NC and anti-miR-29b. (c) Overlap of 5-hmC and 5-mC modified regions in LNCaP and BicR cells. (d) The FOXA1 motif was most enriched in 5-hmC regions (P=1.0 × 10−1878, HOMER55was used for motif analysis and calculation ofPvalue). (e) 5-hmC modification in the vicinity of FOXA1-binding regions. FOXA1-binding sites were determined by ChIP-seq in LNCaP cells. 5-hmC signals around FOXA1 peaks are summarized. (f) Interaction of TET2 with FOXA1. Upper: immunoprecipitation by anti-TET2 antibody. LNCaP cells were treated with 10 nM DHT or vehicle for 24 h. Lysates were immunoprecipitated by an anti-TET2 antibody. Lower: interaction of TET2 with FOXA1 in VCaP cells. VCaP cells were transfected with TET2 expression vector or empty vector for 72 h. Lysates were immunoprecipitated by an anti-FOXA1 antibody or normal IgG. (g) Representative mapping of 5-hmC-, FOXA1-, AR-, K4me1- and K4me3-binding regions in a representative 5-hmC target gene,NKX3.1. (h) FOXA1 enhancer activity is regulated by miR-29 and TET2 pathway. ChIP analysis of AR, K4me1 and FOXA1 in the 3tUTR enhancer region (ARBS) ofNKX3.1. ChIP qPCR was performed to evaluate the enrichment (n=3). Values represent the mean±s.d. *P<0.05, **P<0.01 (two-sided Student’st-test). IB, immunoblot; IP, immunoprecipitation. Figure 6: Global analysis of 5-hmC-regulated pathways in prostate cancer progression. ( a ) Global mapping of genomic regions modified with 5-hmC (upper) and 5-mC (lower) in prostate cancer cells. Genomic DNA was extracted from LNCaP cells and from BicR cells treated with anti-NC or anti-miR-29b. Binding regions were determined by MACS. ( b ) Validation of 5-hmC levels in LNCaP and BicR cells by hMeDIP. Cells were transfected with anti-NC and anti-miR-29b. ( c ) Overlap of 5-hmC and 5-mC modified regions in LNCaP and BicR cells. ( d ) The FOXA1 motif was most enriched in 5-hmC regions ( P =1.0 × 10 −1878 , HOMER [55] was used for motif analysis and calculation of P value). ( e ) 5-hmC modification in the vicinity of FOXA1-binding regions. FOXA1-binding sites were determined by ChIP-seq in LNCaP cells. 5-hmC signals around FOXA1 peaks are summarized. ( f ) Interaction of TET2 with FOXA1. Upper: immunoprecipitation by anti-TET2 antibody. LNCaP cells were treated with 10 nM DHT or vehicle for 24 h. Lysates were immunoprecipitated by an anti-TET2 antibody. Lower: interaction of TET2 with FOXA1 in VCaP cells. VCaP cells were transfected with TET2 expression vector or empty vector for 72 h. Lysates were immunoprecipitated by an anti-FOXA1 antibody or normal IgG. ( g ) Representative mapping of 5-hmC-, FOXA1-, AR-, K4me1- and K4me3-binding regions in a representative 5-hmC target gene, NKX3.1 . ( h ) FOXA1 enhancer activity is regulated by miR-29 and TET2 pathway. ChIP analysis of AR, K4me1 and FOXA1 in the 3tUTR enhancer region (ARBS) of NKX3.1 . ChIP qPCR was performed to evaluate the enrichment ( n =3). Values represent the mean±s.d. * P <0.05, ** P <0.01 (two-sided Student’s t -test). IB, immunoblot; IP, immunoprecipitation. Full size image Surprisingly, we found that the FOXA1 motif was predominantly enriched in the 5-hmC regions ( Fig. 6d ). FOXA1, a central transcription factor of prostate cancer biology, coordinates AR binding and promotes tumour progression [31] , [32] . We observed a significant overlap of the 5-hmC regions with FOXA1-binding regions and K4me1-modified regions ( Fig. 6e ; Supplementary Fig. 15a ). Furthermore, the 5-hmC regions obtained by miR-29b knockdown overlapped with ARBSs throughout the genome ( Supplementary Fig. 15b ). TET2 ChIP-seq signals were observed in the vicinity of 5-hmC sites in LNCaP cells; these were also validated by ChIP analysis ( Supplementary Fig. 16a–e ). Moreover, we demonstrated that TET2 interacts with FOXA1 ( Fig. 6f ; Supplementary Fig. 17 ). For example, in the genomic locus of NK3 homeobox 1 ( NKX3.1 ), an AR collaborative factor [33] , we detected decreased 5-hmC levels in BicR cells and increased 5-hmC levels following anti-miR-29b transfection around FOXA1-bound enhancer region ( Fig. 6g ). Although ChIP analysis revealed that miR-29b inhibition decreases FOXA1 binding, subsequent AR recruitment and enhancer activity, this inhibition was reversed by TET2 knockdown, suggesting the positive and negative roles of miR-29b and TET2 in FOXA1 enhancer activity, respectively ( Fig. 6h ). Conversely, we also observed a positive effect of miR-29b on FOXA1 binding by the addition of miR-29 ( Supplementary Fig. 18a–c ). We also examined whether 5-hmC modifications modify FOXA1 DNA-binding ability. In gel shift assay, FOXA1 interact with DNA probe including FOXA1-binding sequence identified by ChIP-seq in MTOR locus ( Supplementary Fig. 18d ). We observed 5-hmC modification reduced FOXA1 binding in vitro . Thus, 5-hmC modulation could be a crucial epigenetic marker for the negative regulation of AR recruitment or FOXA1 enhancer activity. Impact of 5-hmC modification on global gene regulation We evaluated the effects of 5-hmC on gene regulation by directional RNA sequencing. RefSeq genes associated with 5-hmC are significantly included among those genes upregulated in BicR cells compared with LNCaP cells, suggesting a negative role of 5-hmC in gene expression ( Fig. 7a,b ). Kyoto Encyclopedia of Genes and Genomes pathway enrichment analysis of the upregulated genes revealed that they are associated with various prostate cancer-related pathways such as AR , mammalian target of rapamycin ( mTOR ), signal tranducer and activator of transcription 3 ( STAT3 ) and cell migration ( Fig. 7c ), which are involved in HRPC progression. Interestingly, androgen-mediated regulation of NKX3.1 is enhanced in BicR cells, suggesting AR hypersensitivity, because NKX3.1 is a positive regulator for AR binding ( Fig. 7a ). We found that mTOR [34] is the most enriched signalling pathway among these 5-hmC-regulated genes in AR-positive HRPC cell line ( Fig. 7c,d ). The androgen-mediated induction of MTOR and NKX3-1 genes was inhibited by anti-miR-29b ( Fig. 7e ), indicating that 5-hmC could be an epigenetic marker associated with the repression of the transcriptional activity of AR. Furthermore, androgen-mediated enhancer activity caused by FOXA1-binding was negatively regulated by miR-29b knockdown and reversed by TET2 knockdown ( Fig. 7f ). Furthermore, enhanced mTOR activation at the protein level in BicR or VCaP cells was dependent on miR-29a/b ( Fig. 7g ; Supplementary Fig. 19a ). 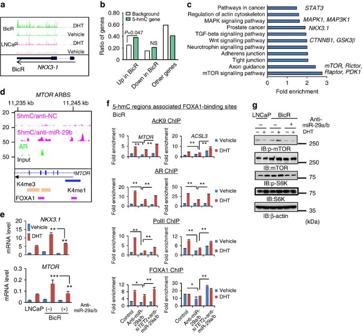Figure 7: Identification of prostate cancer-related genes such asmTORas 5-hmC targets. (a)NKX3.1is upregulated in BicR cells. The RNA-seq view ofNKX3.1locus is shown56. Arrows indicate the direction of transcription. (b) Regulation of expression levels of 5-hmC target genes in BicR cells. 5-hmC-binding genes only in LNCaP cells were selected and changes in their expression levels in BicR cells compared with LNCaP cells are summarized.Pvalue is obtained byχ2-test. NS, not significant. (c) Pathway analysis of 5-hmC-regulated genes. The top 10 pathways are shown. (d) Epigenetic regulation of ARBS in the enhancer region ofMTOR. Mapping of 5-hmC-, FOXA1-, AR-, K4me1- and K4me3-binding regions is shown. (e) LNCaP and BicR cells treated with anti-NC or anti-29a/b were treated with vehicle or 10 nM DHT for 24 h. mRNA levels ofNKX3.1andMTORwere analysed by qRT–PCR (n=3). Values represent the mean±s.d. **P<0.01, ***P<0.001 (two-sided Student’st-test). (f) Two days before androgen stimulation, BicR cells were transfected with anti-NC, anti-miR-29a/b or anti-miR-29a/b+siTET2#1 (1 nM). BicR cells were treated with 10 nM DHT or vehicle for 24 h. ChIP analysis was performed using anti-AcH3K9, pol II, FOXA1 and AR antibodies. Enrichments were measured by qPCR and normalized by an IgG control (n=3). Values represent the mean±s.d. *P<0.05, **P<0.01 (two-sided Student’st-test). (g) Lysates from LNCaP and BicR cells transfected with anti-NC or anti-miR-29a/b were analysed by western blot analysis to detectmTORsignals in prostate cancer. IB, immunoblot. Figure 7: Identification of prostate cancer-related genes such as mTOR as 5-hmC targets. ( a ) NKX3.1 is upregulated in BicR cells. The RNA-seq view of NKX3.1 locus is shown [56] . Arrows indicate the direction of transcription. ( b ) Regulation of expression levels of 5-hmC target genes in BicR cells. 5-hmC-binding genes only in LNCaP cells were selected and changes in their expression levels in BicR cells compared with LNCaP cells are summarized. P value is obtained by χ 2 -test. NS, not significant. ( c ) Pathway analysis of 5-hmC-regulated genes. The top 10 pathways are shown. ( d ) Epigenetic regulation of ARBS in the enhancer region of MTOR . Mapping of 5-hmC-, FOXA1-, AR-, K4me1- and K4me3-binding regions is shown. ( e ) LNCaP and BicR cells treated with anti-NC or anti-29a/b were treated with vehicle or 10 nM DHT for 24 h. mRNA levels of NKX3.1 and MTOR were analysed by qRT–PCR ( n =3). Values represent the mean±s.d. ** P <0.01, *** P <0.001 (two-sided Student’s t -test). ( f ) Two days before androgen stimulation, BicR cells were transfected with anti-NC, anti-miR-29a/b or anti-miR-29a/b+si TET2 #1 (1 nM). BicR cells were treated with 10 nM DHT or vehicle for 24 h. ChIP analysis was performed using anti-AcH3K9, pol II, FOXA1 and AR antibodies. Enrichments were measured by qPCR and normalized by an IgG control ( n =3). Values represent the mean±s.d. * P <0.05, ** P <0.01 (two-sided Student’s t -test). ( g ) Lysates from LNCaP and BicR cells transfected with anti-NC or anti-miR-29a/b were analysed by western blot analysis to detect mTOR signals in prostate cancer. IB, immunoblot. Full size image Microarray analysis in LNCaP cells demonstrated that a greater number of 5-hmC-associated genes were significantly upregulated than downregulated by si TET2 ( Fig. 8a ) when compared with the background, suggesting that TET2 is mainly involved in the gene repression. By combining these results with the RNA sequencing (RNA-seq) analysis, 281 genes were induced by si TET2 and upregulated in BicR, while, 83 genes were repressed ( Supplementary Fig. 20a ). Interestingly, sequences surrounding both the upregulated and downregulated genes presented significant enrichment of FOXA1 and AR-binding sites, suggesting the role of FOXA1 and AR for positive and negative gene regulation caused by TET2 ( Supplementary Fig. 20b,c ). The inhibition or addition of TET2 led to the upregulation or repression of FOXA1-associated androgen-regulated genes, respectively, indicating a negative role of 5-mC hydroxylation in FOXA1-driven enhancer and promoter activity ( Fig. 8b,c ). Importantly, anti-miR-29b-mediated transcriptional repression of androgen-regulated genes was relieved by TET2 knockdown ( Fig. 8d,e ). 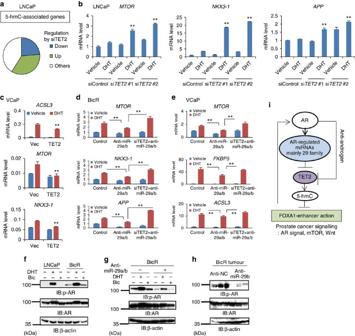Figure 8: Critical role of TET2 in regulating androgen signalling and AR. (a) Knockdown ofTET2induced gene transcription. Microarray analysis was performed to explore the effect of TET2 on gene expression profiles. LNCaP cells were treated with siControl or siTET2#1 (1 nM) for 48 h. (b) AR transcriptional activity is enhanced byTET2knockdown. LNCaP cells were treated with siControl, siTET2#1 or siTET2#2 (1 nM) for 48 h. Cells were treated with vehicle or 10 nM DHT for 24 h. mRNA expression levels were measured by qRT–PCR (n=3). Values represent the mean±s.d. **P<0.01 (two-sided Student’st-test). (c) AR transcriptional activity is repressed by TET2 overexpression. VCaP cells were transfected with a TET2 expression vector (Halo-TET2) or empty vector. After 48-h incubation, cells were treated with vehicle or 10 nM DHT for 24 h. Expression levels of mRNAs were measured by qPCR (n=3). Values represent the mean±s.d. **P<0.01 (two-sided Student’st-test). (d) Reduced expression of miR-29a/b repressed androgen-mediated gene induction. BicR cells were transfected with control, anti-miR-29a/b or anti-miR-29a/b+siTET2#1 (1 nM;n=3). Values represent the mean±s.d. **P<0.01 (two-sided Student’st-test). (e) VCaP cells were transfected with anti-NC, anti-miR-29a/b or anti-miR-29a/b+siTET2#1 (1 nM). After incubation for 72 h, cells were treated with DHT or vehicle for 24 h. Expression levels of androgen-regulated genes were analysed by qRT–PCR (n=3). Values represent the mean±s.d. **P<0.01 (two-sided Student’st-test). (f) Upregulation of p-AR (ser81) in BicR cells in the absence of 10 nM DHT or 10 μM bicalutamide treatment compared with LNCaP cells. LNCaP, BicR, cells were treated with vehicle, 10 nM DHT or 10 μM bicalutamide for 24 h. Western blot analysis was performed to evaluate the protein levels of p-AR. (g) BicR cells were treated with anti-NC or anti-miR-29a/b for 48 h. Cells were treated with vehicle, 10 nM DHT or 10 μM bicalutamide for 24 h. Western blot analysis was performed to evaluate the protein levels of p-AR. (h) Expression level of phosphorylated AR (Ser81) in tumours derived from BicR cells by western blot analysis. (i) Working model of TET2 repression by AR-regulated miRNAs or antagonist-bound AR to control the genome-wide 5-hmC status for prostate cancer progression. IB, immunoblot. Figure 8: Critical role of TET2 in regulating androgen signalling and AR. ( a ) Knockdown of TET2 induced gene transcription. Microarray analysis was performed to explore the effect of TET2 on gene expression profiles. LNCaP cells were treated with siControl or si TET2 #1 (1 nM) for 48 h. ( b ) AR transcriptional activity is enhanced by TET2 knockdown. LNCaP cells were treated with siControl, si TET2 #1 or si TET2 #2 (1 nM) for 48 h. Cells were treated with vehicle or 10 nM DHT for 24 h. mRNA expression levels were measured by qRT–PCR ( n =3). Values represent the mean±s.d. ** P <0.01 (two-sided Student’s t -test). ( c ) AR transcriptional activity is repressed by TET2 overexpression. VCaP cells were transfected with a TET2 expression vector (Halo-TET2) or empty vector. After 48-h incubation, cells were treated with vehicle or 10 nM DHT for 24 h. Expression levels of mRNAs were measured by qPCR ( n =3). Values represent the mean±s.d. ** P <0.01 (two-sided Student’s t -test). ( d ) Reduced expression of miR-29a/b repressed androgen-mediated gene induction. BicR cells were transfected with control, anti-miR-29a/b or anti-miR-29a/b+si TET2 #1 (1 nM; n =3). Values represent the mean±s.d. ** P <0.01 (two-sided Student’s t -test). ( e ) VCaP cells were transfected with anti-NC, anti-miR-29a/b or anti-miR-29a/b+si TET2 #1 (1 nM). After incubation for 72 h, cells were treated with DHT or vehicle for 24 h. Expression levels of androgen-regulated genes were analysed by qRT–PCR ( n =3). Values represent the mean±s.d. ** P <0.01 (two-sided Student’s t -test). ( f ) Upregulation of p-AR (ser81) in BicR cells in the absence of 10 nM DHT or 10 μM bicalutamide treatment compared with LNCaP cells. LNCaP, BicR, cells were treated with vehicle, 10 nM DHT or 10 μM bicalutamide for 24 h. Western blot analysis was performed to evaluate the protein levels of p-AR. ( g ) BicR cells were treated with anti-NC or anti-miR-29a/b for 48 h. Cells were treated with vehicle, 10 nM DHT or 10 μM bicalutamide for 24 h. Western blot analysis was performed to evaluate the protein levels of p-AR. ( h ) Expression level of phosphorylated AR (Ser81) in tumours derived from BicR cells by western blot analysis. ( i ) Working model of TET2 repression by AR-regulated miRNAs or antagonist-bound AR to control the genome-wide 5-hmC status for prostate cancer progression. IB, immunoblot. Full size image Furthermore, Cyclin-dependent kinase 1 (CDK1), a 5-hmC-regulated gene, is involved in AR phosphorylation (Ser81) in response to DHT stimulation [35] . The CDK1 is upregulated in BicR cells and repressed by the inhibition of miR-29a/b ( Supplementary Fig. 19b,c ). Consistent with this result, a high p-AR (Ser81) level was observed in BicR cells without DHT, and this level was dependent on the miR-29a/b expression ( Fig. 8f,g ). Moreover, bicalutamide-dependent repression of p-AR observed in LNCaP cells is found to be diminished in BicR cells ( Supplementary Fig. 19d ). We found that the p-AR enhancement in BicR tumours with bicalutamide or in other AR-positive cell lines is inhibited by miR-29a/b knockdown ( Fig. 8h and Supplementary Fig. 19e–g ). Taken together, our results suggest that miR-29-mediated TET2 repression activated 5-hmC targeting AR regulators such as CDK1 and then increase AR sensitivity. The present study establishes a genome-wide map of the 5-hydroxymethylome in prostate cancer cells and reveals the oncogenic role of decreased 5-hmC levels in the comprehensive modulation of signalling pathways involved in prostate cancer progression ( Fig. 8i ). In the present study, we demonstrate that TET2 is repressed by androgen using CAGE. We also present a novel mechanism that TET2 repression by androgen is mediated by miRNA induction. In addition, AR ChIP-seq analysis in HRPC cells indicates that antagonist-bound AR directly represses the TET2 -enhancer activity by modifying histones. Short RNA sequence analysis revealed a strong androgen-mediated induction of members of the miR-29 family, which in turn repress the expression of TET2 to promote prostate tumour growth. We also found that the androgen antagonist, bicalutamide, differentially regulates TET2 expression in hormone-dependent and HRPC cells, suggesting a possible involvement of TET2 in anti-androgen withdrawal syndrome, a frequent clinical complication [36] . Recent research demonstrates that the dysregulation of miRNA expression profiles contributes to the pathogenesis of human malignancies [37] , [38] , [39] , [40] . Because the expression of the miR-29 family is reduced in several cancer tissues as compared with normal tissues, the role of the miR-29 family in cancer is controversial [41] , [42] . While the precise role of the miR-29 family members in cancer is still unclear, they are known to promote metastasis in breast cancer [43] , [44] . Importantly, our clinical study of prostate cancer samples demonstrates that miR-29 is negatively correlated with TET2 and highly expressed in cancers with poor prognoses. We have shown, using both in vitro and in vivo studies, that the miR-29 family is a key determinant of the progression of prostate cancer to HRPC. In vitro , miR-29 family members promote the cell proliferation and migration of HRPC cells by activating cell motility and cell cycle-associated gene expression. Furthermore, miR-29a/b depletion enhanced the TET2 expression and repressed castration-resistant cell growth. In vivo , the miR-29 family members enhance AR antagonist- or castration-resistant tumour growth. These results denote a significant oncogenic role of miR-29 in prostate cancer progression. Our findings indicate a novel epigenetic role of AR-dependent TET2 repression in the FOXA1 cistrome. We demonstrated that 5-hmC modifications are enriched among global FOXA1-binding sites and inhibit FOXA1 binding at specific loci. However, it would be important to confirm genome-wide FOXA1-binding sites were modulated by miR-29a/b or TET2 by ChIP-seq in the future study. In addition, this research highlights the importance of global gene regulation by the miR-29 family in determining cancer cell fate. Identification of the signalling pathways regulated by 5-hmC would facilitate the elucidation of the mechanisms responsible for prostate cancer progression. We show that the hydroxylation of 5-mC inhibits the expression of p-AR, mTOR and oncogenic proteins such as STAT [45] and Wnt [46] , which are involved in the signalling pathways that govern the progression of prostate cancer to HRPC. Collectively, our results identify 5-hydroxymethylation, rather than methylation alone, as the primary target of the miR-29 family members in prostate cancer cells. Interestingly, genes in the mTOR-related pathway were most enriched in areas encoding the components of 5-hmC-regulated signalling pathways. We identified the MTOR gene as a typical example of such a gene cluster and as a novel androgen target, particularly in HRPC. Several AR- and FOXA1-binding sites were identified in the intron region of MTOR via ChIP-seq. The hydroxylation of 5-mC at ARBSs was repressed in HRPC cells and enhanced by inhibition of miR-29 expression. Our results indicate that loss of 5-hmC at ARBSs increased FOXA1 enhancer activity for MTOR induction by androgen. Recent studies have demonstrated the importance of mTOR in prostate cancer metastasis and its potential use as a target for HRPC therapy [34] , [47] . Our results raise the possibility that acquired AR hypersensitivity could promote HRPC tumour growth. The hydroxylation of 5-mC by inhibition of miR-29 expression suppressed AR-dependent gene expression, and TET2 inhibition reversed the effect of miR-29 inhibition on AR signalling and cell growth. Mechanistically, the modulation of FOXA1 enhancer activity by TET2 repression could promote AR recruitments. We also found the expression level of one AR-collaborating factor, NKX3-1, which is encoded by a highly androgen-sensitive gene, was also affected by 5-hmC. Moreover, we showed that CDK1 is one of the 5-hmC-targeted genes in prostate cancer cells and is upregulated in HRPC cells. We also noted that phosphorylation of AR at serine 81 is promoted by miR-29 induction in HRPC cells. Phosphorylation of AR at serine 81 by CDK1 has been reported to increase AR sensitivity by promoting AR binding to specific ARBSs [35] . Thus, on the basis of the results of our clinical and biological experiments, we demonstrate the significance of TET regulation for the progression to HRPC by activating AR sensitivity. In conclusion, our results indicate that TET2 signalling play an important role in the FOXA1 cistrome transcriptional network by controlling the global epigenetic code, 5-hmC, during prostate cancer progression. This finding highlights the importance of 5-hmC as a key epigenetic marker that regulates the steroid hormone activity by modulating FOXA1 binding. In addition, we also revealed a novel divergent function of miR-29 as a crucial epigenetic regulator that represses TET2 in cancer progression. Thus, developing novel epigenetic approaches for inhibiting miR-29 or modifying TET2-mediated pathway may have important implications for treating advanced prostate cancer. HeliScope CAGE The majority of transcriptome protocols running on second-generation sequencing platforms have relied on two PCR steps, one for pre-amplification of complementary DNA (cDNA) and the other for clonal amplification of templates on the flow cell before sequencing. To avoid any potential bias in the identification and quantification of RNA molecules, we used single-molecule sequencers for CAGE to identify and quantify the 5′-ends of capped RNAs based on cap trapping. Known genes and alternative promoters were determined after genome mapping. HeliScope CAGE quantifies gene expression with the least variability suggesting its reproducibility [22] , [23] . Total RNA was extracted from LNCaP and BicR cells using ISOGEN (Nippon Gene, Tokyo, Japan). The quality of the total RNA was determined using an Agilent Bioanalyzer, and the RNA integrity number was confirmed to be 9.0 or higher. First-strand cDNA synthesis was performed using SuperscriptIII (Life Technologies) and random primer. Oxidized cDNA/RNA hybrids were biotinylated for cap trapping. After poly(dA) tailing, sequencing with the HeliScope Single Molecule Sequencer was performed according to the manufacturer’s manual [22] . Gene expression was measured with the number of reads aligned within a 500-bp distance from the RefSeq transcript 5p-ends, where their genomic coordinates were downloaded from the UCSC Genome Browser database. The read counts were normalized to tags per million based on the total number of aligned reads in the human genome reference. All CAGE tags with one or more overlapping base pair were grouped on the same strand into a single tag cluster (TC). To analyse the androgen-regulated transcriptional program, we prepared total RNA extracted from LNCaP cell lines treated with 10 nM R1881 at seven time points in each biological duplicate. In contrast to previous CAGE studies by the Genome sequencer FLX system (454) [48] , we observed 57% of the signals within 500 bp of the 5′-ends of messenger RNAs based on the genomic coordinates of the reference full-length transcripts of RefSeq. We aggregated neighbouring CAGE tags on the genome into TCs and obtained 19,644 TCs. Of these, 8,309 (43%) fell outside of the RefSeq gene promoters. By analysing gene expression at each time point, we identified sets of genes regulated by androgen treatment using strict threshold for significance ( P value<0.01, Fisher’s exact test, Q -value<0.01). RNA sequencing RNA-seq library construction and sequencing were performed according to the manufacturer’s protocol for the Applied Biosystems SOLiD 3 Plus System (Applied Biosystems). The library was sequenced using SOLiD Opti Fragment Library Sequencing kit Master Mix 50 chemistry (Applied Biosystems), which gives 50-bp readings. The RNA-seq readings were analysed using whole-transcriptome software tools from Applied Biosystems. Matching locations were subsequently used to generate counts for annotated features, exons, transcripts or genes using RefSeq Genes to determine the exons genomic locations of known transcripts or coverage files (wiggle format). Finally, genes expression was determined as the number of reads per kilobase of exon model per million mapped reads. Genome-wide methylation and 5-hydroxymethylation analysis Enrichment of methylated DNA (5-mC) was performed using a Methyl Collector Ultra kit (Active Motif). Briefly, genomic DNA was sheared by sonication. The sheared DNA was incubated with a His-tagged recombinant MBD2b/MBD3L1 protein complex. These protein–DNA complexes were captured with nickel-coated magnetic beads. Enrichment of 5-hydroxymethylated DNA (5-hmC) was performed using a Hydroxymethyl Collector kit (Active Motif), which utilizes a β-glucosyltransferase enzyme to transfer a modified glucose moiety to 5-hydroxymethylcytosine residues in double-stranded DNA. This modified glucose was then used to chemically attach a biotin conjugate to facilitate capture and enrichment with streptavidin magnetic beads. Enriched double-stranded DNA was sequenced by a Hiseq 2000 Genome Analyzer (Illumina) applying the ChIP-seq method. Sequence readings were mapped onto the human genome (hg18) using the CASAVA software. The 5-mC and 5-hmC-enriched regions were identified by calculating P value and FDR using MACS [30] ) and the threshold was P <10 −5 and FDR<0.01. The 5-hmC peaks were annotated to human RefSeq genes and the genes with 5-hmC peaks in the promoter or gene-body regions were chosen for further analysis. ChIP sequencing AR and TET2 ChIP-seq was performed using an Illumina Genome Analyzer (Illumina, San Diego, CA, USA). Libraries were prepared according to the manufacturer’s instructions. Unfiltered 36-bp sequence readings were aligned to the human reference genome (hg18) using CASAVA v1.7 (Illumina). Signal scores and P value for AR-binding sites was calculated by MACS. The threshold of binding sites was P value<10 −5 . Integrative genomic viewer version 2.2 was used for visualization. hMeDIP hMeDIP analysis was performed using a hMeDIP kit (Active Motif) according to the manufacturer’s instructions. Briefly, genomic DNA was sonicated by a Bioruptor sonicator (Cosmobio). The sonicated DNA fragments (1 μg of each sample, length<500 bp) were denatured and diluted by the immunoprecipitation buffer. The diluted DNA was incubated with 4 μl of anti-5-hmC antibody (Active Motif) at 4 °C overnight. Antibody–DNA complexes were captured by protein A/G beads, and the enriched 5-hmC-containing DNA fragments were purified. We quantified the enrichment of 5-hmC by quantitative PCR (qPCR). DNA dot blot analysis Genomic DNA was extracted from cells using a DNeasy kit (Qiagen). Denatured DNA was spotted on a nitrocellulose membrane (Waterman) and crosslinked by ultraviolet irradiation. Briefly, the membrane was first blocked with 5% milk in TBS–Tween 20 for 1 h and then incubated with an anti-5-hmC or 5-mC antibody (1:10,000; Active Motif) for 1 h. Following which, the membrane was incubated with a horseradish peroxidase-conjugated anti-rabbit IgG antibody (Beyond Time) for 1 h at room temperature, washed three times with TBS–Tween 20, and finally the DNA was visualized using enhanced chemiluminescence kit (GE-Healthcare). Immunohistochemistry Formalin-fixed tissues were embedded in paraffin and sectioned. A Histofine kit (Nichirei, Tokyo, Japan), which employs the streptavidin–biotin amplification method, was used for immunohistochemical analysis of TET2, 5-mC and 5-hmC. The antigen–antibody complex was visualized with a 3,3′-diaminobenzidine solution (1 mM 3,3′-diaminobenzidine, 50 mM Tris-HCl buffer (pH 7.6) and 0.006% H 2 O 2 ). During immunohistochemical analysis, immunoreactivity was evaluated in >1,000 carcinoma cells in each case, and the percentage of immunoreactivity (labelling index) was determined by certified pathologists. Cases with the labelling index of >10% were considered TET2-, 5-mC- or 5-hmC-positive carcinoma in this study. miRNA in situ hybridization (ISH) MiRNA ISH Buffer and Controls kit (Exiqon, Woburn, MA, USA) was used for ISH in this study according to the manufacturer’s protocol. Briefly, tissue specimens were fixed with 10% formalin and embedded in paraffin. Slides were deparaffinized and incubated with proteinase-K (10 μg ml −1 ) for 10 min at 37 °C. The hybridization mixture, containing 20 nM double-DIG LNA miRNA probe for miR-29a, miR-29b or scramble-miR (Exiqon), was applied and hybridized for 1 h at 60 °C. The probe sequences used in this study were as follows: miR-29a, 5′-TAACCGATTTCAGATGGTGCTA-3′; mR-29b, 5′-AACACTGATTTCAAATGGTGCTA-3′; and scramble-miR, 5′-GTGTAACACGTCTATACGCCCA-3′. Slides were incubated with RNase (20 μg ml −1 , Wako Pure Chemical Industries, Osaka, Japan) for 30 min at 37 °C, and anti-digoxigenin-AP Fab fragments (1:1,000, Roche) were applied as the primary antibody. NBT/BCIP solution (Roche) was used for visualization and then the slides were counterstained with Nuclear Fast Red. Short RNA sequencing Purified short RNAs were ligated to chimeric oligonucleotide adaptors and reverse transcribed to cDNA. PCR products with a size of 11–40 nt were eluted from 12% polyacrylamide gels. The PCR products were digested by a restriction enzyme, concatenated, column purified to eliminate short concatemers and sequenced using an Illumina/Solexa GAIIx Genome Sequencer (Illumina, San Diego, CA, USA). RNAs were aligned to the human genome (NCBI build 35) and were used to search for miRNA sequences in the miRBase 9.1 database. We selected sequences with a single match in the best BLAST hits. miRNA quantitative PCR Total RNA was extracted using a mirVana miRNA Isolation Kit (Ambion). RNA (10 ng) was reverse transcribed to cDNA using a TaqMan miRNA reverse transcription kit (Applied Biosystems). QPCR for cDNA was performed using TaqMan miRNA assay primers and a StepOne Real-Time PCR System (Applied Biosystems). The relative level of miRNA was calculated by normalizing the target gene signal by the signal for U6B small nuclear RNA. Plasmid construction To overexpress TET2, we purchased a Halo-tagged expression vector, which included the TET2 cDNA clone (TET2a: FHC22012 and TET2b: FHC22011) from Promega. A TET2 -3′UTR sequence containing the miR-29-binding sites or a subsequent sequence lacking these sites was generated by PCR amplification using the following primers: TET2 -3′UTR-F: 5′-GGGCTCGAGAGTATTACAGTGACAGGAAT-3′, TET2 -3′UTR-R: 5′-CCCGCGGCCGCATATTTGTAGCAGGCTGAGT-3′ and TET2 -3′UTR-NC-F: 5′-GGGCTCGAGATCATAATGTGAGCTAAGAA-3′, TET2 -3′UTR-NC-R: 5′-CCCGCGGCCGCCAGTTTAACAAATGACAGTA-3′. Amplified sequences were cloned into the psiCHECK-2 vector (Promega). Vectors were designated as TET2 -3′UTR-Luc and TET2 -3′UTR-NC-Luc, respectively. Cell culture and reagents VCaP and 293T cells were grown in DMEM medium supplemented with 10% fetal bovine serum (FBS), 50 U ml −1 penicillin and 50 μg ml −1 streptomycin. 22Rv1, DU145, RWPE and LNCaP cells were grown in RPMI medium supplemented with 10% FBS, 50 U ml −1 penicillin and 50 μg ml −1 streptomycin. LTAD cells were grown in phenol red-free RPMI medium supplemented with 10% charcoal–dextran-stripped FBS, 50 U ml −1 penicillin and 50 μg ml −1 streptomycin. BicR cells were grown in RPMI medium supplemented with 10% FBS, 10 μM bicalutamide, 50 U ml −1 penicillin and 50 μg ml −1 streptomycin. LNCaP cells were obtained from American Type Culture Collection. Short tandem repeat (STR) analysis was performed for the authentication of the cell lines, which were newly established from LNCaP cells or provided from other laboratories (VCaP, Du145 and RWPE). We also checked the expression patterns of AR and its variants to verify the prostate cancer cell lines. Cells were routinely checked for mycoplasma contamination using Mycoplasma Detection Kit (JENA Bioscience GmbH, Jena, Germany). We used cells verified to be mycoplasma free for experiments. The antibodies used in this study were 5-hmC, 5-mC (Active Motif), TET2 (Abcam), mTOR (Cell Signaling), p-mTOR (Cell Signaling), S6K (Cell Signaling), p-S6K (Cell Signaling), p-AR (Ser81; Millipore), AR (Santa Cruz Biotechnology), FOXA1 (Abcam), EZH2 (BD Biosciences), RNA pol II (Millipore), AcH3 (Millipore), H3K4me3, H3K4me1, H3K9me2 (Abcam), Halo (Promega) and β-actin (Sigma). ChIP and quantitative PCR For ChIP using AR, FOXA1 and TET2 antibody, cells were crosslinked with 1% formaldehyde for 10 min and stopped by adding 0.2 M glycine. Cells were lysed by lysis buffer [48] , [49] and chromatin DNA was sheared by sonication. Sonicated lysates were incubated overnight at 4 °C with specific antibodies. Then, protein G agarose beads were added and rotated for 2 h. The beads were washed several times and incubated at 65 ° overnight to reverse crosslink. DNA was purified with ethanol precipitation. The fold enrichment relative to the IgG-IP control or % of input was quantified by qPCR using SYBR Green PCR master mix and the ABI StepOne System (Life Technologies, Carlsbad, CA, USA). We used GAPDH locus as a negative control (NC) [48] . The primer sequences for the detection of ARBSs by qPCR are listed in Supplementary Table 6 . qRT–PCR Total RNA was isolated using the ISOGEN reagent. First-strand cDNA was generated using a PrimeScript RT reagent kit (Takara, Kyoto, Japan). The primer sequences are listed in Supplementary Table 6 . Expression levels were quantified by qPCR [48] , [49] using SYBR Green PCR master mix and the ABI StepOne system (Life technologies). Western blot analysis Whole-cell lysates were prepared using NP40 lysis buffer. Protein concentration was determined by the BCA assay (Pierce, Rockford, IL, USA). Each protein lysate was loaded onto 8 or 10% SDS–polyacrylamide gels, separated by electrophoresis and electrotransfered onto Immobilon-P Membranes (Millipore, Billerica, MA, USA). Membranes were incubated with primary antibodies overnight and then incubated with secondary antibodies. Antibody–antigen complexes were detected using ECL Western Blotting Substrate (Pierce). Films were quantified by scanning densitometry using Image J software (NIH). All full-scan images of immunoblotting are shown in Supplementary Fig. 21 . Luciferase assay LNCaP cells were incubated with phenol red-free medium supplemented with 5% dextran–charcoal-stripped FBS for 24 h before transfection. Cells were transfected with pGL3 vectors including ARBSs and tk-pRL using the FuGENE HD reagent (Promega, Madison, WI, USA). Twenty-four hours after transfection, the cells were treated with 10 nM DHT or vehicle for 24 h, and then luciferase activity was determined using luminometer [49] . Migration assay Cellular migration assays were performed using a 24-well plate matrigel-coated invasion chambers (BD Biosciences, San Jose, CA, USA). Briefly, cells (5 × 10 4 cells) were suspended in serum-free RPMI medium and then transferred into suspended inserts with 8 μm pores. RPMI medium with 10% FBS was placed at the bottom of the wells and the cells were cultured for 24 h. Invading cells were fixed with methanol and stained with Giemsa [50] . The number of invading cells in five random fields was counted using a microscope, and the average number of cells per field was calculated. EMSA Gel shift assay was performed using the DIG Gel shift kit (Roche) with DIG-labelled oligonucleotides containing FOXA1-binding sites (in the MTOR locus) identified by ChIP-seq. HA-tagged FOXA1 protein was overexpressed in 293T cells and purified using an anti-HA antibody. After mixing probes with FOXA1 protein at room temperature, samples were analysed on a 6% polyacrylamide gel electrophoresis gel. After transferring to a positive-charged nylon membrane (Roche), signals were detected using an anti-DIG antibody (Roche). 5-mC- and 5-hmC-modified oligonucleotides were purchased from Eurosins Genomics (Tokyo, Japan). The oligonucleotide sequence for preparing the probe was as follows: 5′-CCTAGGTTGTTTACAAACACAGAATGCTTG-3′. 3C assay 3C assay was basically performed as previously described [51] . Briefly, crosslinked samples were incubated with HindIII restriction enzyme at 37 °C overnight and then incubated with T4 DNA ligase (Promega) at 16 °C for 4 h. Samples were diluted and immunoprecipitated with AR antibody at 4 °C overnight. Next, the samples were rotated with protein A agarose beads for 2 h at 4 °C. The beads were washed with ChIP dilution buffer and de-crosslinked. Primer sequences used for PCR amplifications were as follows: promoter, 5′-CTTCTCTTATGCCGCGAAACT-3′ and enhancer, 5′-GTCACTGGGATTCATGCAAA-3′. siRNA transfection For siRNA experiments, we purchased Stealth RNAi siRNAs (Life Technologies) targeting TET2 (#1: HSS123253 and #2:HSS123254), EZH2 (HSS176652) [52] , AURKA (HSS186148), HBP1 (HSS178254) and a negative control siRNA. Cells were transfected with siRNAs using siGene (Promega) 48–72 h before each experiment. miRNA and anti-miRNA transfection Transfection of small RNAs pre-miRNA 29a/b, anti-miRNA-29a/b, control miRNA (NC) and anti-negative control (anti-NC; purchased from Life Technologies) were performed using siPort transfection reagent (Life Technologies) according to the manufacturer’s protocol with some modifications as described in the Supplementary Table 7 or Figure legends. Patients and tissue samples We obtained 102 prostate cancer samples from patients who underwent a radical prostatectomy performed at the University of Tokyo Hospital (Tokyo, Japan). The Tokyo University Ethics Committee approved this study, and informed consent was obtained from each patient before surgery. The ages of the patients ranged from 52 to 78 years (mean, 67 years), and pretreatment serum prostate-specific antigen levels ranged from 1.2 to 136 ng ml −1 (mean, 16.9 ng ml −1 ). The prostate tissue sections submitted for this study contained 95 benign and 102 cancerous foci. The sections were evaluated by two specialized pathologists (T.S. and K.-i.T.). Clinicopathological parameters such as Gleason scores, pathological primary tumour (pT) stages and pathological regional lymph node (pN) stages were summarized in Supplementary Table 2 . Thirty-three patients were treated with surgery alone. The remaining patients, who had pT3 cancer and/or experienced a postoperative prostate-specific antigen nadir of >0.2 ng ml −1 , received adjuvant androgen deprivation and/or radiation therapy. Patients were followed up by their surgeons at 3-month intervals for 5 years and yearly thereafter. The mean patient follow-up period was 144±56 months (range: 10–240 months). Cell proliferation assay Cells were plated at 3 × 10 3 cells per well in 96-well plates. For RNA interference experiments, cells were transfected with siRNA 24 h after plating. The MTS [3-(4,5-dimethylthiazol-2-yl)-5-(3-carboxymethoxyphenyl)-2-(4-sulfophenyl)-2H-tetrazolium, inner salt] assay was performed using the CellTiter 96 Aqueous MTS reagent (Promega) according to the manufacturer’s instructions. The experiment was performed in quintuplicate. In vivo tumour formation assay LNCaP, BicR, 22Rv1 and LTAD (3 × 10 6 ) cells were subcutaneously injected into each side of twenty 5-week-old male BALB/C nude mice. For the experiment of LNcaP and BicR xenografts, the mice were randomly divided into three groups when the tumour volumes reached 100 mm 3 . Each group was treated with vehicle or bicalutamide (20 mg kg −1 ; Santa Cruz Biotechnology) orally every other day and an intratumoral injection of anti-miRNA-29b was started. To study the effect of miR-29a/b knockdown on castration-resistant tumour growth, 22Rv1 and LTAD xenografts were grown. Once the tumours reached 100 mm 3 , mice were physically castrated and randomly divided into two groups. Each group was treated with an intratumoral injection of anti-miRNA-29a/b or anti-NC. Each tumour was injected with 5 μg of anti-miR-29b, a/b or anti-NC, 3 times a week using Lipofectamine RNAi MAX Transfection Reagent (Life Technologies). Tumour volume was determined using the following formula: V =0.5 × r 1 × r 2 × r 3 ( r 1< r 2< r 3). Tokyo university animal ethics committee approved these experiments. Microarray For expression microarrays, a GeneChip Human Exon 1.0 ST Array (Affymetrix, Santa Clara, CA, USA) was used according to the manufacturer’s protocol. Data analysis was performed using the Affymetrix Microarray Suite software. To compare arrays, normalization was performed on data from all probe sets. GO term and Pathway analysis was performed using DAVID [53] , [54] . Statistical analyses For cell line experiments, statistical differences ( P values) among groups were obtained using the two-sided Student’s t -test. All experiments were performed at least twice and similar results were obtained. P values <0.05 were considered statistically significant. Statistical analysis was performed using Graphpad Prism 5 software (GraphPad Software, San Diego, CA, USA) or MS Excel. The association between miRNA expressions and clinicopathological factors was evaluated using the Student’s t -test, Wilcoxon signed rank test, cross-table using the χ 2 -test, Spearman rank correlation test or the correlation coefficient ( R ) and regression equation. We excluded samples if the obtained values were more than twice the s.d. of the mean. For xenograft experiments, sample sizes were calculated using s.d in the preliminary experiments and the expected difference of two groups. Other sample sizes were equal or greater than the recommended minimum sample size in the past publications. A cancer-specific survival curve was generated according to the Kaplan–Meier method, and statistical significance was calculated using the log-rank test. Accession codes. The microarray, CAGE, RNA-seq and ChIP-seq data have been deposited in Gene Expression Omnibus ( GSE66039 ). We also used previously deposited data ( GSE62492 , GSE58428 and GSE58309 (refs 50 , 52 , 56 )). How to cite this article: Takayama K. et al. TET2 repression by androgen hormone regulates global hydroxymethylation status and prostate cancer progression. Nat. Commun. 6:8219 doi: 10.1038/ncomms9219 (2015).